Redox-responsive self-healing materials formed from host–guest polymers Expanding the useful lifespan of materials is becoming highly desirable, and self-healing and self-repairing materials may become valuable commodities. The formation of supramolecular materials through host–guest interactions is a powerful method to create non-conventional materials. Here we report the formation of supramolecular hydrogels and their redox-responsive and self-healing properties due to host–guest interactions. We employ cyclodextrin (CD) as a host molecule because it is environmentally benign and has diverse applications. A transparent supramolecular hydrogel quickly forms upon mixing poly(acrylic acid) (pAA) possessing β-CD as a host polymer with pAA possessing ferrocene as a guest polymer. Redox stimuli induce a sol−gel phase transition in the supramolecular hydrogel and can control self-healing properties such as re-adhesion between cut surfaces. High-performance materials such as stimulus-responsive and maintenance-free self-healing materials [1] , [2] , [3] , [4] , [5] , [6] , [7] , [8] , [9] have attracted much attention due to modern environmental and energy concerns. Recently developed functional soft materials possessing switching, self-healing and self-repairing features are expected to have diverse applications (for example, in architectural materials and external coatings). Some research groups have attempted to create switching soft materials such as remotely actuated nanomaterials [10] , [11] , [12] , [13] , [14] , artificial molecular muscles [15] , [16] , drug-delivery systems [17] , [18] , biosensors and shape memory materials. Although there are previous examples of supramolecular hydrogels [19] where a sol−gel phase transition occurs using heat [20] , pH [21] , light [22] , [23] , [24] , [25] or redox [26] , [27] , [28] , [29] , [30] , [31] , [32] as a stimulus, it is difficult to create multi-functional soft materials owing to complicated designs and syntheses. Hence, redox stimulus-responsive self-healing materials have yet to be reported. Previously, we have reported stimulus-responsive supramolecular materials possessing host and guest polymers [33] , [34] , [35] . Supramolecular materials consisting of host and guest polymers have unique features due to selective complementary interactions. Host–guest interactions are versatile, and can be used to prepare supramolecular materials, which have easily tuned switching efficiencies and functions. Self-healing and self-repairing properties may be achieved using supramolecular materials that consist of host and guest polymers. The duality of supramolecular materials, which possess both switching and self-healing properties, has attracted both supramolecular chemists and materials scientists. Here, we report supramolecular materials using poly(acrylic acid) (pAA; M w =25×10 4 ) modified with cyclodextrins (pAA-CDs) [36] as a host polymer and pAA with ferrocene (pAA-Fc) as a guest polymer. Ferrocene (Fc) derivatives have attracted attention due to their redox-responsive properties. Variations in the redox potential can induce a reversible sol−gel phase transition in a supramolecular hydrogel formed by pAA-6βCD and pAA-Fc. Moreover, supramolecular materials formed by host–guest interactions exhibit self-healing and self-repairing properties. 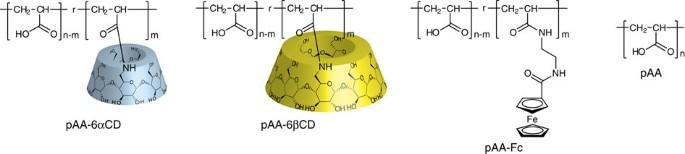Figure 1: Chemical structures of the host polymers and the guest polymer. Host polymers (pAA-6αCD and pAA-6βCD), and the guest polymer (pAA-Fc) were synthesized by side-chain modification of pAA. Preparation of host and guest polymers Figure 1 depicts the chemical structures of the host polymers (pAA-CDs) and a guest polymer (pAA-Fc). pAA-CDs were prepared by the reaction of amino-CDs (6-amino-αCD and 6-amino-βCD) with pAA ( Supplementary Fig. S1 ). According to 1 H nuclear magnetic resonance (NMR) spectroscopy, amino-CDs were substituted into 4−5% of the carboxylic acid groups of pAA ( Supplementary Fig. S2 and Supplementary Table S1 ). These host polymers are called pAA-6αCD and pAA-6βCD for substitutions by 6-amino-αCD and 6-amino-βCD, respectively. pAA-Fc was prepared by the reaction of aminoethylamide Fc with pAA ( Supplementary Fig. S3 ), and Fc was substituted into 2.7% of the carboxylic acid groups of pAA ( Supplementary Fig. S4 and Supplementary Table S1 ). Figure 1: Chemical structures of the host polymers and the guest polymer. Host polymers (pAA-6αCD and pAA-6βCD), and the guest polymer (pAA-Fc) were synthesized by side-chain modification of pAA. 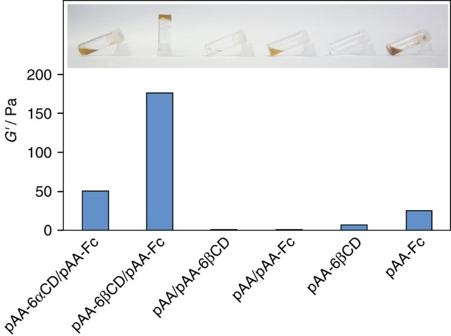Figure 2: Values of storage elastic modulus. pAA-6αCD/pAA-Fc, pAA-6βCD/pAA-Fc, pAA/pAA-6βCD, pAA/pAA-Fc, pAA-6βCD and pAA-Fc (2 wt%) in a pH 9 buffer solution. Insets are photographs of hydrogelation between host polymers and guest polymers (2 wt%) in aqueous solutions. Although a 1:1 mixture of a solution of pAA-6αCD/pAA-Fc, pAA-3αCD/pAA-Fc, pAA-3βCD/pAA-Fc, pAA/pAA-6βCD or pAA/pAA-Fc showed the low viscosity, the mixed solution of pAA-6βCD/pAA-Fc selectively increased the viscosity. A hydrogel consisting of pAA-6βCD/pAA-Fc is produced by the complementarity between the β-CD and Fc units. Full size image Hydrogelation between host and guest polymers Figure 2 shows photographs of hydrogelation between the host polymers and a guest polymer (2 wt%) in a pH 9 boric acid/KCl/NaOH buffer solution. The 1:1 mixture of a 2 wt% solution of pAA-6αCD/pAA-Fc, pAA/pAA-6βCD or pAA/pAA-Fc in an aqueous solution had a negligible effect on the viscosity. On the other hand, the mixed solution of pAA-6βCD/pAA-Fc selectively increased the viscosity of the solution to yield a hydrogel ( Supplementary Movie 1 ). These results indicate that not only the host–guest complementarity but also multipoint crosslinks have important roles in forming the supramolecular hydrogel. Figure 2: Values of storage elastic modulus. pAA-6αCD/pAA-Fc, pAA-6βCD/pAA-Fc, pAA/pAA-6βCD, pAA/pAA-Fc, pAA-6βCD and pAA-Fc (2 wt%) in a pH 9 buffer solution. Insets are photographs of hydrogelation between host polymers and guest polymers (2 wt%) in aqueous solutions. Although a 1:1 mixture of a solution of pAA-6αCD/pAA-Fc, pAA-3αCD/pAA-Fc, pAA-3βCD/pAA-Fc, pAA/pAA-6βCD or pAA/pAA-Fc showed the low viscosity, the mixed solution of pAA-6βCD/pAA-Fc selectively increased the viscosity. A hydrogel consisting of pAA-6βCD/pAA-Fc is produced by the complementarity between the β-CD and Fc units. Full size image Figure 2 shows storage elastic moduli ( G′ ) for pAA-6αCD/pAA-Fc, pAA-6βCD/pAA-Fc, pAA/pAA-6βCD, and pAA/pAA-Fc, pAA-6βCD, and pAA-Fc (1+1 wt%) in pH 9 buffer solutions, respectively. Although other samples exhibited G′ <50 Pa, pAA-6βCD/pAA-Fc had the highest elasticity (176 Pa), which was more than thrice the value of the comparison cases. 2D NOESY NMR confirmed the interactions between β-CD and pAA-Fc ( Supplementary Fig. S5 ) and between the β-CD moieties of pAA-6βCD and pAA-Fc ( Supplementary Fig. S6 ). Previous studies have suggested that the association constant of Fc in its reduced state for β-CD is larger than that for αCD (Fc/αCD; K a =0.14×10 3 M −1 , Fc/βCD; K a =17×10 3 M −1 ) [37] , [38] . The K of β-CD for the Fc group of pAA-Fc was 1.1×10 3 M −1 , which is suitable for a competitive host molecule for the Fc group of pAA-Fc. ( Supplementary Figs S7 and S8 ). To clarify the complementarity between β-CD and the Fc groups (reduced state), competitive guest or host molecules were added to the pAA-6βCD/pAA-Fc hydrogel (2 wt%). Adamantane carboxylic acid sodium salt (AdCANa) was used as a competitive guest, because the association constant for β-CD ( K a =35×10 3 M −1 ) [39] is higher than that of Fc. Adding AdCANa (10 eq. for the βCD group of pAA-6βCD) into the pAA-6βCD/pAA-Fc hydrogel led to a sharp decrease in the elasticity from 176 Pa to 23.3 Pa to form the sol state ( Supplementary Fig. S9a ). Similarly, adding β-CD (10 eq. for the Fc group of pAA-Fc) as a competitive host into the pAA-6βCD/pAA-Fc hydrogel induced a phase transition into the sol state ( Supplementary Fig. S9b ). They inhibited the formation of an inclusion complex between the β-CD unit of pAA-6βCD and the Fc unit of pAA-Fc. Next, we examined the effects of the host–guest ratio on the elasticity change. The elasticity of pAA-6βCD/pAA-Fc was estimated by varying the ratio of pAA-6βCD and pAA-Fc in the monomer unit equivalent. Although pAA-6βCD/pAA-Fc in the non-equivalent ratio demonstrated moderate elasticities, the 1:1 ratio of pAA-6βCD/pAA-Fc displayed the largest G′ value (176 Pa) ( Supplementary Fig. S10 ). These results indicate that a hydrogel consisting of pAA-6βCD/pAA-Fc is produced by the extensive complementarity between the β-CD and Fc units. Redox-responsive sol−gel switching We investigated the effect of the redox reagents on the phase transition of the pAA-6βCD/pAA-Fc hydrogel. We chose NaClO aq. (14 mM) as an oxidant and glutathione (GSH) as a reductant. Adding NaClO aq. (0.1 ml) to the pAA-6βCD/pAA-Fc hydrogel (0.4 ml) decreased the viscosity, transforming the hydrogel into the sol. 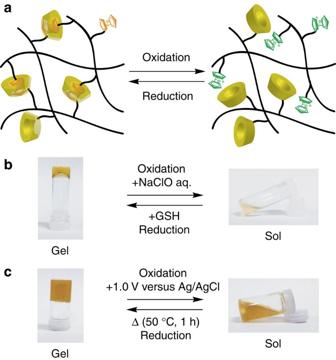Figure 3: Redox-responsive sol−gel transition experiment. (a) Schematic illustration of sol−gel transition. (b) Sol−gel transition experiment using chemical reagents. Adding NaClO aq. to the pAA-6βCD/pAA-Fc hydrogel induced a phase transition into the sol state, and continuous addition of GSH to the sol recovered the elasticity to yield the hydrogel again. (c) Sol−gel transition experiment using electrochemical reactions. Electrochemical oxidation (+1.0 V versus Ag/AgCl) transformed the hydrogel into the sol, whereas reduction recovered the viscosity, reverting it back to the hydrogel. In contrast, continuous addition of GSH (1.2 mg) to the sol recovered the elasticity, reverting it back to the hydrogel ( Figure 3b ). β-CD showed a high affinity for the reduced state of the Fc group due to its hydrophobic nature, whereas the oxidized state of the Fc group (Fc + ) exhibited a low affinity for β-CD due to the cationic Fc + group [40] . Figure 3: Redox-responsive sol−gel transition experiment. ( a ) Schematic illustration of sol−gel transition. ( b ) Sol−gel transition experiment using chemical reagents. Adding NaClO aq. to the pAA-6βCD/pAA-Fc hydrogel induced a phase transition into the sol state, and continuous addition of GSH to the sol recovered the elasticity to yield the hydrogel again. ( c ) Sol−gel transition experiment using electrochemical reactions. Electrochemical oxidation (+1.0 V versus Ag/AgCl) transformed the hydrogel into the sol, whereas reduction recovered the viscosity, reverting it back to the hydrogel. Full size image Next, we attempted to electrochemically control the pAA-6βCD/pAA-Fc hydrogel. The pAA-6βCD/pAA-Fc hydrogel was electrolyzed with a potentiostat using a three-electrode system (platinum plate (working), platinum wire (counter) and Ag/AgCl electrode (reference)) and 50 mM of NaBr as a supporting electrolyte. Electrochemical oxidation of the pAA-6βCD/pAA-Fc hydrogel decreased the elasticity, and consequently transformed the hydrogel into the sol. Subsequent reduction by heating the sol at 50 °C recovered the elasticity, yielding the hydrogel ( Fig. 3c ; Supplementary Fig. S11 ). The redox reactions between Fc (reduced state) and Fc + in its oxidized state were tracked by ultraviolet–visible ( Supplementary Figs S12-S15 ) and circular dichroism spectroscopies ( Supplementary Fig. S16 ). A mixture of pAA-6βCD ([βCD]=2 mM) and Fc carboxylic acid (FcCOOH, 2 mM) exhibited a d−d transition band around 400−450 nm, but the band disappeared upon oxidation with NaClO aq. Before oxidizing, the circular dichroism spectra exhibited a negative Cotton band around 400−450 nm, which was assigned to the induced Cotton band between the Fc group and β-CD on the side chain of pAA-6βCD in an aqueous solution. Adding NaClO as an oxidant decreased the band, indicating that oxidized Fc is not included in the cavity of β-CD. Consequently, both chemical and electrochemical redox reactions for the pAA-6βCD/pAA-Fc hydrogel yield reversible sol−gel phase transitions. Self-healing property of pAA-6βCD/pAA-Fc hydrogel We speculated that the pAA-6βCD/pAA-Fc hydrogel would exhibit a self-healing property because a characteristic feature of the pAA-6βCD/pAA-Fc hydrogel is the reversible host–guest interaction between the side chains of both polymers. Thus, we conducted a break test during continuous step strain measurements. As a precondition of the pAA-6βCD/pAA-Fc hydrogel for the break test, we confirmed that the hydrogel did not relax ( G′ > G′′ ) in the frequency range 0.01−100 rad·s −1 , which was characterized by dynamic viscoelastic measurements ( Supplementary Figs S17 and S18 ). Supplementary Figure S19 demonstrates that the morphology of the pAA-6βCD/pAA-Fc hydrogel remained the same for over 72 h. We measured the rheological property of the pAA-6βCD/pAA-Fc hydrogel (1+1 wt%) under small (0.1%) and large (200%) strains ( Supplementary Fig. S20 ). Under a 0.1% strain, G′ was larger than G′′ , indicating that the pAA-6βCD/pAA-Fc hydrogel formed a self-standing hydrogel. However, the G′ and G′′ values were inverted under 200% strain, indicating that the pAA-6βCD/pAA-Fc hydrogel was converted into the sol state. We assumed that the interaction between the β-CD and Fc units was cutoff by the 200% strain in the sol state of pAA-6βCD/pAA-Fc. When placed under 0.1% strain, G′ and G′′ returned to their original values. G′ of the pAA-6βCD/pAA-Fc sol recovered to 90% of its initial state in 20 s, and the hydrogel was observed in 500 s. This recovery behaviour was repeatable for at least three cycles of varying strains. The reason that the pAA-6βCD/pAA-Fc sol transformed to the hydrogel is because the inclusion complex between the βCD and Fc units was reconstructed under 0.1% strain, suggesting that the characteristic self-healing property of pAA-6βCD/pAA-Fc hydrogel is formed by a host–guest interaction. Macroscopic self-healing of pAA-6βCD/pAA-Fc hydrogel Based on this rheological property, we confirmed the self-healing ability of the pAA-6βCD/pAA-Fc hydrogel. A cube-shaped pAA-6βCD/pAA-Fc hydrogel (1+1 wt%) was cut in half using a razor edge, and then rejoined ( Fig. 4a ). After standing for 24 h, the crack disappeared, and the sample hydrogel sufficiently healed to form one gel. To demonstrate the complementary host–guest interaction between the β-CD and the Fc groups, competitive guest and host molecules were added to the cut plane of the pAA-6βCD/pAA-Fc hydrogel ( Supplementary Fig. S21 ). A 3 mM solution of AdCANa as the competitive guest, β-CD as the competitive host or D -glucose as a reference sample was placed on the cut surfaces, and then the two gels were reattached. After 24 h, the samples with a competitive guest or host did not heal, whereas the sample with D -glucose healed regardless of the amount of D -glucose added. These results indicate that the self-healing property is due to the Fc and β-CD moieties, which form an inclusion complex on the cut surfaces of hydrogels. The adhesive strength of the two gels was confirmed by the wedge-shaped strain compression test ( Supplementary Fig. S22 ). After the two gels were rejoined for 24 h, the adhesion strength on the joint surface reached a steady value, indicating that the interaction of the Fc and β-CD moieties achieved equilibrium on the surface. The adhesion strength on the joint surface recovered 84% of the initial gel's strength after 24 h ( Supplementary Fig. S23 ). 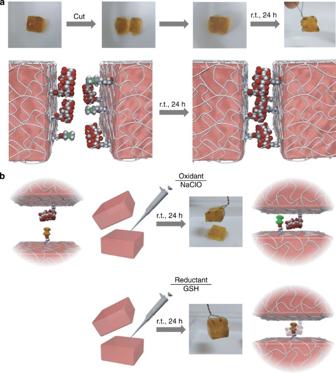Figure 4: Self-healing experiments. (a) After standing for 24 h, two cut pAA-6βCD/pAA-Fc hydrogel (1+1 wt%) pieces were rejoined, and the crack sufficiently healed to form one gel. (b) Redox-responsive healing experiment of the pAA-6βCD/pAA-Fc hydrogel using oxidizing/reducing agents. A pAA-6βCD/pAA-Fc hydrogel (2 wt%) was cut in half, and NaClO aq. was spread on the cut surface. After 24 h, healing was not observed. Re-adhesion was observed 24 h after spreading GSH aq. onto the oxidized cut surface. Figure 4: Self-healing experiments. ( a ) After standing for 24 h, two cut pAA-6βCD/pAA-Fc hydrogel (1+1 wt%) pieces were rejoined, and the crack sufficiently healed to form one gel. ( b ) Redox-responsive healing experiment of the pAA-6βCD/pAA-Fc hydrogel using oxidizing/reducing agents. A pAA-6βCD/pAA-Fc hydrogel (2 wt%) was cut in half, and NaClO aq. was spread on the cut surface. After 24 h, healing was not observed. Re-adhesion was observed 24 h after spreading GSH aq. onto the oxidized cut surface. Full size image Controlling self-healing ability by redox reaction Finally, we investigated the control of the self-repairing property of the pAA-6βCD/pAA-Fc hydrogel by redox stimuli. A pAA-6βCD/pAA-Fc hydrogel (2 wt%) was cut in half, and the cut surfaces were coated with an aqueous solution of NaClO (7 mM, 20 μl). Then the two pieces were reattached according to the experimental operation shown in Figure 4b . After 24 h, healing was not observed. The NaClO-applied gels did not form an inclusion complex between the β-CD and Fc + units. However, the surface re-adhered after spreading GSH aq. (20 mM, 20 μl), a reducing agent, onto the oxidized cut surface and allowing the gel to stand for 24 h. We successfully realized reversible sol−gel switching and a self-healing supramolecular hydrogel system consisting of pAA-6βCD/pAA-Fc. Although microscale switching of supramolecular complexes by redox is well known, a macroscale morphological change is difficult to achieve. This work demonstrates that intelligent supramolecular hydrogels may be formed using a main chain with a sufficient length and an adequate number of guest molecules to generate reversible multipoint crosslinks between pAA-6βCD/pAA-Fc. A redox reaction alters the morphology of a supramolecular hydrogel by controlling the formation of an inclusion complex. These stimulus-responsive self-healing properties are similar to the selective cell-adhesive protein observed on a cellular surface. Stimulus-responsive self-healing properties have many general applications. Thus, we believe that these stimulus-responsive and healing properties may eventually be used in stimulus-responsive drug-delivery carriers and peripheral vascular embolization materials with healing properties that target cancer cells and myoma. Materials Poly(acrylic acid) (pAA, M w =250,000) and D 2 O were obtained from Wako Pure Chemical Industries, Ltd. α-Cyclodextrin and β-cyclodextrin were obtained from Junsei Chemical Co., Ltd. Triethylamine (Et 3 N), ethylenediamine, sodium hydroxide, potassium hydroxide, boric acid, potassium chloride and sodium hypochlorite aqueous solution were obtained from Nacalai Tesque Inc. Benzotriazol-1-yl-oxytripyrrolidinophosphonium hexafluorophosphate (PyBOP), 3-amino-3-deoxy-α-cyclodextrin and 3-amino-3-deoxy-β-cyclodextrin, ferrocenecarboxylic acid, adamantanecarboxylic acid and oxalyl chloride were obtained from Tokyo Kasei Inc. Glutathione was obtained from KOHJIN Co., Ltd. DMSO- d 6 was obtained from Merck & Co., Inc. A highly porous synthetic resin (DIAION HP-20) used for column chromatography was purchased from Mitsubishi Chemical Co., Ltd. Dialytic tube (MWCO=14,000) was purchased from Sanko Junyaku Inc. Water used for the preparation of the aqueous solutions (except for NMR measurements) was purified with a Millipore Elix 5 system (Millipore). Other reagents were used without further purification. Measurements The 1 H NMR and 2D NMR (NOESY) spectra were recorded at 500 MHz with a JEOL JNM-ECA 500 NMR spectrometer (JEOL). Chemical shifts were referenced to the solvent values ( δ =2.49 p.p.m. for dimethylsulphoxide and δ =4.79 p.p.m. for HOD). The ultraviolet–visible absorption spectra were recorded with a JASCO V-650 and a Hitachi U-4100 spectrometer in water with 1 cm quartz cell at room temperature. Circular dichroism spectra and ultraviolet-visible spectra were recorded on a JASCO J820 spectrometer in water with 1 cm quartz cell at room temperature. Dynamic viscoelasticity was measured using an Anton Paar MCR301 rheometer (Anton Paar). Mechanical properties of the gel were measured by the mechanical tension testing system (Rheoner, RE-33005, Yamaden Ltd.). Preparation and characterization of pAA-CDs Poly(acrylic acid) ( M w =250,000) was dissolved in 20 ml of N,N -dimethylformamide (DMF). To this solution, PyBOP (0.06 eq. of acrylic acid unit) and Et 3 N (0.06 eq. of acrylic acid unit) were added. After stirring for 2 h, a mono-amino-mono-deoxy-CD was added, and the solution was stirred for another 12 h at room temperature. The polymer product was reprecipitated from 200 ml of ethanol and washed with ethanol. The polymer was dissolved in water, and dialyzed for 12 days with a dialytic tube (MWCO=14,000). After dialysis, each pAA–CD was obtained by freeze–drying. pAA-6αCD; 1 H NMR (500 MHz, pD 9 buffer, 30°C): δ 1.56 to 2.12 (C H 2 (pAA)), 2.31–2.65 (C H (pAA)), 3.61–3.80 (C 2,4 H (CD)), 3.80–4.11 (C 3,5,6 H (CD)), 5.00–5.23 (C 1 H (CD)). pAA-6βCD; 1 H NMR (500 MHz, pD 9 buffer, 30°C): δ 1.56–2.12 (C H 2 (pAA)), 2.31–2.65 (C H (pAA)), 3.61–3.80 (C 2,4 H (CD)), 3.80–4.10 (C 3,5,6 H (CD)), 5.05–5.22 (C 1 H (CD)). Synthesis and characterization of Fc-CONH-(CH 2 ) 2 -NH 2 Ferrocenecarboxylic acid of 2.00 g (8.7 mmol) was suspended in 120 ml of dichloromethane (DCM). Then 2 ml (23.3 mmol, 2.7 eq.) of oxalyl chloride was added dropwise, and the suspension was stirred for 3 h at room temperature. The orange suspension turned into a red solution. After evaporating the solvent, ferrocenecarboxyl chloride (red solid) was dissolved in 60 ml of DCM. A volume of 6 ml (89.9 mmol, 10 eq.) of ethylenediamine was dissolved in 60 ml of DCM, and the ferrocenecarboxyl chloride solution was added dropwise. After stirring overnight at room temperature, the solution was washed with 80 ml of 10% KOH aq., and the DCM layer was collected and evaporated. The orange solid was washed with 300 ml of hexane: ethyl acetate=9:1, and the solid product was collected via a centrifuge and dried for 4 days at 50 °C to obtain Fc-CONH-(CH 2 ) 2 -NH 2 as a yellow powder in 83% yield. 1 H NMR (500 MHz, D 2 O, 30 °C): δ 2.90 (2 H, t, Fc-CONH-CH 2 -C H 2 -NH 2 ), 3.46 (2 H, t, Fc-CONH-C H 2 -CH 2 -NH 2 ), 4.36 (5 H, s, Cp), 4.61 (2 H, t, Cp), 4.89 (2 H, t, Cp). Synthesis and characterization of pAA-Fc PyBOP (0.22 g, 0.42 mmol, 0.06 eq. of acrylic acid unit) was added to a 40 ml DMF solution of pAA ( M av =250,000, 500.3 mg). In all, 0.95 g (0.35 mmol, 0.05 eq. of acrylic acid unit) of Fc-CONH-(CH 2 ) 2 -NH 2 was dissolved in 10 ml of DMF, and 0.06 ml (0.43 mmol, 0.06 eq. of acrylic acid unit) of Et 3 N was added. This solution was added dropwise to the pAA solution and stirred for 12 h at room temperature. After stirring, the solution was diluted with water and dialyzed in water for 7 days with dialytic tube (MWCO=14,000). After dialysis, pAA-Fc was obtained by freeze–drying. 1 H NMR (500 MHz, pD 9 buffer, 30 °C): δ 1.40–1.91 (C H 2 (pAA)), 2.05–2.50 (C H (pAA)), 4.37 (s, Cp), 4.61 (s, Cp), 4.91 (s, Cp (overlapped with HOD)). Breaking stress measurement of the pAA-6βCD/pAA-Fc hydrogel One centimetre cube-shaped pAA-6βCD/pAA-Fc hydrogel (3 wt%) was cut in half using a razor edge, and then rejoined at 24°C (waiting time <5 min.). After standing for 24 h, the breaking stress was measured by a creep metre with a wedge-shaped plunger ( Supplementary Figs S22 and S23 ). How to cite this article: Nakahata, M. et al . Redox responsive self-healing materials formed from host–guest polymers. Nat. Commun. 2:511 doi: 10.1038/ncomms1521 (2011).